Non-Darwinian dynamics in therapy-induced cancer drug resistance The development of drug resistance, the prime cause of failure in cancer therapy, is commonly explained by the selection of resistant mutant cancer cells. However, dynamic non-genetic heterogeneity of clonal cell populations continuously produces metastable phenotypic variants (persisters), some of which represent stem-like states that confer resistance. Even without genetic mutations, Darwinian selection can expand these resistant variants, which would explain the invariably rapid emergence of stem-like resistant cells. Here, by using quantitative measurements and modelling, we show that appearance of multidrug resistance in HL60 leukemic cells following treatment with vincristine is not explained by Darwinian selection but by Lamarckian induction. Single-cell longitudinal monitoring confirms the induction of multidrug resistance in individual cells. Associated transcriptome changes indicate a lasting stress response consistent with a drug-induced switch between high-dimensional cancer attractors. Resistance induction correlates with Wnt pathway upregulation and is suppressed by β-catenin knockdown, revealing a new opportunity for early therapeutic intervention against the development of drug resistance. The development of resistance to chemotherapy and target-selective drugs is the prime cause of therapy failure [1] . Mechanisms implicated range from the canonical ‘acquisition’ of a resistant cell phenotype to whole-tumour level changes involving non-neoplastic stroma [2] , [3] . Cell-level resistance is still considered the major cause of loss of drug sensitivity, because it can readily be reproduced in cell cultures and explained by the nature of associated molecular changes, such as the expression of detoxification proteins [4] , structural alteration of the drug target protein [5] or activation of alternative growth and survival pathways [6] , [7] , [8] . One of the best characterized molecular mechanisms of cellular resistance is the expression of ABC-transporter family proteins, such as multidrug resistance protein 1 (MDR1), which pumps a variety of drugs out of the cell [9] , thereby conferring the MDR phenotype. But how are these molecular changes acquired? Current paradigm holds that treatment selects for cancer cells carrying a random genetic mutation that pre-exists before treatment and happens to confer a survival advantage in the presence of the drug, resulting in the ‘emergence’ of drug-resistant clones [10] , [11] . Point mutations in drug target proteins that alter the drug docking site [5] or genomic rearrangements in the MDR1 regulatory region [12] , [13] that cause high expression of the MDR1 protein support the theory of a somatic evolution of cancer cells that follows the Darwinian scheme of mutation and selection. However, the increasing realization that cancer cells exhibit a rich intraclonal dynamics manifest as ‘non-genetic heterogeneity’ complicates the picture [14] . Such phenotype heterogeneity in the absence of genetic variation is the combined consequence of multistability in gene expression dynamics (the coexistence of multiple stable steady states, or ‘attractors’, in gene regulatory networks [15] , [16] , [17] ) and of gene expression noise [18] . Thus, one genome can produce multiple enduring (stable) or transient (metastable) phenotypic states. This departure from the simple one-to-one mapping between genotype and phenotype necessitates a re-examination of the standard scheme of somatic evolution driven by random genetic mutations [19] , [20] . Non-genetic cell state dynamics that is manifest in the behaviour of tumour cells has recently received renewed interest and is best understood in terms of stochastic multi-attractor dynamics: tumour cells within a clonal population spontaneously switch between several (meta)stable attractor states, which represent different developmental states, including mesenchymal, epithelial, as well as cancer stem-cell-like states [21] , [22] , [23] , [24] , [25] , [26] . Cells in the latter state are naturally endowed with increased xenobiotics resistance [22] , [27] . In an unperturbed cell population, multistability is manifested as a broad quasi-continuous or as a multimodal distribution of a phenotypic marker across the entire population [15] . Switching between attractor states can occur in two ways: in a spontaneous and stochastic manner [2] because of noise-induced attractor state transition [28] , [29] , and in a directed way following a perturbation by external signals that alter gene expression. Both have consequences for resistance development [30] . First, stochastic non-genetic phenotype switching can act as a source of random variability—the substrate for Darwinian selection [31] , [32] ; cells that by chance occupy states that are more resilient to cytotoxic stress, including therapy-induced cytotoxicity, can be transiently selected for during treatment. As these cell states are non-genetically inherited over many cell generations, they can, in principle, promote evolution according to the Darwinian scheme—in the absence of mutations [29] , [33] . The transient selection of cells in the resistant state allows a subpopulation of temporarily ‘fitter’ cells to expand, thereby increasing the probability for adaptive genetic mutations. Such ‘mutationless preselection’ could accelerate classical Darwinian evolution of drug resistance [31] , [32] , [33] as observed for antibiotic resistance in microorganisms (‘persisters’) [34] , [35] , [36] . Second, induction of attractor state switching by external signals opens the possibility for a Lamarckian scheme of evolution [37] ; a perturbation by cytotoxic agents may ‘instruct’ the cell to enter an attractor state that confers the stem-like, more stress-resistant phenotype—perhaps recapitulating a generic, physiological stress-response—which can be passed on to subsequent cell generations. The non-genetic inheritance of an acquired adaptive trait at the cellular, not organismal level does not violate the neo-Darwinian dogma [37] , [38] , [39] . In fact, chemotherapy and irradiation appear to ‘cause’ the emergence of resistant, stem-like or mesenchymal cancer cells [26] , [40] , [41] , [42] , [43] , [44] , [45] , [46] , [47] , [48] . Promoter analyses have shown that chemotherapy leads to changes in DNA methylation and histone modification in the MDR1 gene locus [49] . Such findings are compatible with both schemes, Darwinian selection and Lamarckian instruction. However, a distinction is rarely explicitly articulated. Although clinicians often take the apparent ‘induction’ of resistance markers following treatment for granted, even viewing it as a form of ‘active’ adaptation because of their rapid and nearly inevitable occurrence, biological orthodoxy assumes by default a Darwinian selection [11] , [21] . The rapid appearance of stemness markers or MDR1 expression following treatment has typically been assessed at the level of tumour tissues or whole-cell populations [43] . Thus, it remains open to what extent the increase of MDR1 expression after treatment is the result of very rapid selection of cells already residing in a state with an active MDR1 locus (Darwinian scheme) or of cell-autonomous gene induction in individual cells (Lamarckian scheme). To understand the elementary dynamics of resistance development, here we determine the relative contribution of these two (non-genetic) schemes of emergence of the MDR phenotype in HL60 acute myeloid leukemia cells, which have long served as a model for MDR1-dependent drug resistance [50] . We show by quantitative measurement and modelling that appearance of MDR1-positive cells 1–2 days after treatment with vincristine (VINC) is predominantly mediated by cell-individual induction of MDR1 expression and not by the selection of MDR1-expressing cells. We confirm this by single-cell longitudinal monitoring. Drug-induced resistance and MDR1 expression correlated with upregulation of Wnt-signalling pathway and could be suppressed by knockdown of β-catenin. Following transient low-dose chemotherapy, surviving cells exhibited a persistent transcriptome change indicative of a lasting stress-response state, consistent with switching between high-dimensional cancer attractors [51] . Acknowledging that resistance can be promoted by a non-genetic Lamarckian mechanism opens a new window for pharmacological interference with resistance. Spontaneous non-genetic drug-resistant state in tumour cells We observed that within a clonally derived population of cultured leukemia cells (HL60 cell line), a small subpopulation (~1–2%) of cells consistently expresses high levels of MDR1 (MDR1 High ) on its cell surface and exhibits the MDR phenotype as measured by the fluorescent dye efflux assay (efflux High ) in the absence of drugs ( Fig. 1a ). The MDR1 Low and MDR1 High subpopulations also differed greatly in their sensitivity to killing by the chemotherapeutic agent VINC [52] ( Fig. 1b ). Both subpopulations correspond to metastable epigenetic states [15] , [53] ( Supplementary Fig. S1 ), because they both re-established the initial population distribution after isolation by fluorescence-activated cell sorting (FACS; Fig. 1a ). The MDR1 Low cells accomplished the repopulation of the original distribution within <1 day, whereas the MDR1 High cells took ~18 days to do so ( Supplementary Fig. S2 ). Similar relaxation dynamics was observed when the functional MDR phenotype was measured using the efflux of fluorescent dyes. 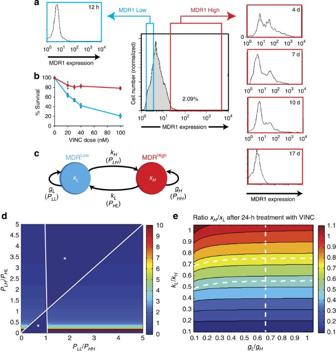Figure 1: Dynamical heterogeneity of MDR1 expression within a clonal population of HL60 cells. (a) A distinct subpopulation of 1–2% of the cells of a clonally derived HL60 cell population consistently expresses high levels of MDR1 on the cell surface in the absence of drug exposures. The MDR1High(red) and MDR1Lowsubpopulations (blue) differ in sensitivity to vincristine after 48 h. (b) Measurements of population dynamics and effective growth were obtained in three different laboratories using different culture of HL60 cells and representative results are shown. Error bar are s.d. of one representative experiment withn=2 biological replicates. (c) Scheme of the state transition model for distinguishing between drug-induced shifts in state transition rates (cell-individual switch to the MDR phenotype) versus drug-induced growth rate differences (selection of the MDR phenotype).x, population fraction of cells in the respective state indicated by the index:H, MDRHigh(effluxHigh) andL, MDRLow(=effluxLow);k, kinetic rate constant for the first-order state transition represented by the arrows.P-state transition probability used in the Markov model. (d) Results of the steady-state Markov model. The state transition and ‘self-renewal’ probabilities required to reach the steady state, shown as heat map with colours indicating the steady-state ratioxH/xL(colour bar) as a function of the ratios of the Markov model probabilitiesP(see Methods section). Change in ratio of transition probabilitiesPLH/PHL(vertical axis) visibly affectsxH/xL, whereas change in the ratioPLL/PHHdoes not result in significant change ofxH/xL. *Undefined regions. (e) Results of the non-equilibrium ODE model. Colour map represents the parameter space, indicating which combination of the two sets of parameters, the ratio of the relative growth rate constants,gL/gH(horizontal axis), and the ratio of the state transition rate constants,kL/kH(vertical axis), causes which population fractionxH/xL(colour map) 24 h after addition of the VINC. Figure 1: Dynamical heterogeneity of MDR1 expression within a clonal population of HL60 cells. ( a ) A distinct subpopulation of 1–2% of the cells of a clonally derived HL60 cell population consistently expresses high levels of MDR1 on the cell surface in the absence of drug exposures. The MDR1 High (red) and MDR1 Low subpopulations (blue) differ in sensitivity to vincristine after 48 h. ( b ) Measurements of population dynamics and effective growth were obtained in three different laboratories using different culture of HL60 cells and representative results are shown. Error bar are s.d. of one representative experiment with n =2 biological replicates. ( c ) Scheme of the state transition model for distinguishing between drug-induced shifts in state transition rates (cell-individual switch to the MDR phenotype) versus drug-induced growth rate differences (selection of the MDR phenotype). x , population fraction of cells in the respective state indicated by the index: H , MDR High (efflux High ) and L , MDR Low (=efflux Low ); k , kinetic rate constant for the first-order state transition represented by the arrows. P -state transition probability used in the Markov model. ( d ) Results of the steady-state Markov model. The state transition and ‘self-renewal’ probabilities required to reach the steady state, shown as heat map with colours indicating the steady-state ratio x H /x L (colour bar) as a function of the ratios of the Markov model probabilities P (see Methods section). Change in ratio of transition probabilities P LH /P HL (vertical axis) visibly affects x H /x L , whereas change in the ratio P LL / P HH does not result in significant change of x H /x L . *Undefined regions. ( e ) Results of the non-equilibrium ODE model. Colour map represents the parameter space, indicating which combination of the two sets of parameters, the ratio of the relative growth rate constants, g L / g H (horizontal axis), and the ratio of the state transition rate constants, k L / k H (vertical axis), causes which population fraction x H / x L (colour map) 24 h after addition of the VINC. Full size image When cells were treated with low-dose VINC (10 nM), within 48 h the MDR1 High subpopulation increased from <2% to >25% in a dose-dependent manner ( Supplementary Fig. S3 ). Appearance of efflux High (MDR) cells was even more rapid and pronounced, typically reaching 30–40% within 24–48 h ( Fig. 2a ). A similar MDR response could be induced with another drug, doxorubicin ( Supplementary Fig. S4 ). This rapid response, in line with prior biochemical analyses [54] , raises the question whether this population shift was driven by a cell-individual induction of the MDR phenotype or by (non-genetic) selection of the pre-existing ‘epigenetic’ MDR1 High cells in the stationary populations because of their survival advantage in the presence of VINC ( Fig. 1b ). In the absence of the drug, the sorted cells in the MDR1 Low /efflux Low state had an ~5-fold net growth advantage over cells in the MDR1 High /efflux High state ( Supplementary Fig. S5 ) and, accordingly, the DNA content of live-cell measurement revealed a smaller fraction of the MDR1 High /efflux High cells in the S/G2 state of the cell cycle ( Supplementary Fig. S6 ). This difference in cell cycle status disappeared when the two subpopulations re-equilibrated to the same MDR1 distribution ( Supplementary Fig. S6 ). In the presence of VINC (10 nM), the relative fitness was reversed: the efflux Low cells exhibited reduced growth and were growth-arrested after 3 days while the efflux High cells survived, displaying slow net population growth ( Supplementary Fig. S5 ). 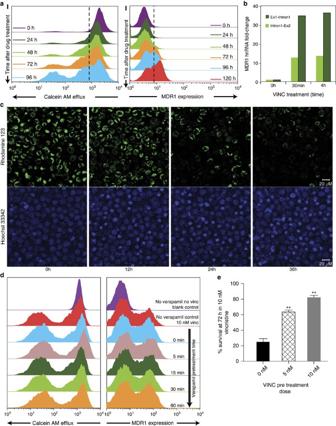Figure 2: Chemotherapy induces expression of the MDR1 protein and the MDR phenotype in HL60 cell population. (a) Flow cytometry measurements of surface MDR1 (immunostaining) and cell efflux capacity (fluorescent dye ejection) at the population level reveal the kinetics for the appearance of the MDR1Highand the MDRHigh/effluxHighsubpopulation following VINC treatment. (b) Quantitative (real-time) RT–PCR (qPCR) using primers targeting the first two exon–intron junctions of MDR1 to measure hnRNA as marker of ongoing transcription. Bar height indicates the average (n=2) of one experiment representative of two independent experiments. The s.d. of all shown qPCR Ct-values was <0.7. (c) Cell-individual induction of the MDR phenotype by VINC. Cells loaded with the fluorescent dye Rh123 (green) as the marker of efflux capacity and stained with a DNA dye (Hoechst 33342, blue) as the cell indicator and to monitor cell death were treated with VINC (10 nM) timet=0 h and were followed by video microscopy under incubator conditions for 36 h. Scale bar, 20 μm (Supplementary Movies 1 and 2for longitudinal tracking of the individual cells andSupplementary Fig. S8). Snapshots at the indicated times are shown. Disappearance of the green fluorescent dye in the viable cells indicates cell-autonomous induction of the MDR phenotype. Nuclear condensation in the Hoechst 33342 stain reveals apoptotic cells. As dying cells will eventually release the dye, we quantified only live cells for dye elimination. After 48 h monitoring of a typical time course, 63% of the live cells treated with VINC exhibited elimination of the dye, representing the switch to the effluxHighphenotype compared with 16% of untreated cells (n=80 cells counted). (d) Saturating doses of verapamil, an inhibitor of MDR1-mediated transport, given at varying times before VINC treatment as indicated, does not alter the induction of MDR1 after 72 h of treatment with VINC. (e) HL60 cells previously exposed for 48 h to the indicated doses (5 nM and 10 nM) of VINC exhibited improved survival compared with naive cells when challenged with 10 nM VINC for 72 h. Error bar, s.d. (n=3), **P<0.01, Student’st-test. Figure 2: Chemotherapy induces expression of the MDR1 protein and the MDR phenotype in HL60 cell population. ( a ) Flow cytometry measurements of surface MDR1 (immunostaining) and cell efflux capacity (fluorescent dye ejection) at the population level reveal the kinetics for the appearance of the MDR1 High and the MDR High /efflux High subpopulation following VINC treatment. ( b ) Quantitative (real-time) RT–PCR (qPCR) using primers targeting the first two exon–intron junctions of MDR1 to measure hnRNA as marker of ongoing transcription. Bar height indicates the average ( n =2) of one experiment representative of two independent experiments. The s.d. of all shown qPCR Ct-values was <0.7. ( c ) Cell-individual induction of the MDR phenotype by VINC. Cells loaded with the fluorescent dye Rh123 (green) as the marker of efflux capacity and stained with a DNA dye (Hoechst 33342, blue) as the cell indicator and to monitor cell death were treated with VINC (10 nM) time t =0 h and were followed by video microscopy under incubator conditions for 36 h. Scale bar, 20 μm ( Supplementary Movies 1 and 2 for longitudinal tracking of the individual cells and Supplementary Fig. S8 ). Snapshots at the indicated times are shown. Disappearance of the green fluorescent dye in the viable cells indicates cell-autonomous induction of the MDR phenotype. Nuclear condensation in the Hoechst 33342 stain reveals apoptotic cells. As dying cells will eventually release the dye, we quantified only live cells for dye elimination. After 48 h monitoring of a typical time course, 63% of the live cells treated with VINC exhibited elimination of the dye, representing the switch to the efflux High phenotype compared with 16% of untreated cells ( n =80 cells counted). ( d ) Saturating doses of verapamil, an inhibitor of MDR1-mediated transport, given at varying times before VINC treatment as indicated, does not alter the induction of MDR1 after 72 h of treatment with VINC. ( e ) HL60 cells previously exposed for 48 h to the indicated doses (5 nM and 10 nM) of VINC exhibited improved survival compared with naive cells when challenged with 10 nM VINC for 72 h. Error bar, s.d. ( n =3), ** P <0.01, Student’s t -test. Full size image Quantitative model of cell state interconversion The current paradigm in tumour biology assumes a predominantly selection-based mechanism to explain population-level shifts of phenotypes, even for acquisition of epigenetic states [21] , [55] . This process requires that the spontaneous presence of 1–2% cells in the MDR1 High /efflux High state ( Fig. 1a ) exploit their growth advantage in the presence of VINC ( Supplementary Fig. S5 ). To quantify the theoretical contribution of selection versus instruction ( Fig. 1c ), we analysed the observed relative growth and induction kinetics in two mathematical models. First, we used a simple kinetic state transition Markov model to examine the contribution of growth rate and transition rate in a population at steady state as often employed for modelling tumour cell dynamics [21] (Methods). With the observed numbers for the ratio of the observed effective growth rate constants ( g L , g H ; Table 1 ), we found that a stationary state with a proportion of 1.5% efflux High cells, as observed, does not exist unless one accepts substantial state transitions between the efflux High and efflux Low states ( Fig. 1d ). Consequently, already under basal conditions (absence of drugs) the measured difference in the effective growth rates of the two subpopulations in isolation is far from being able to ensure the preservation of the observed steady proportions of these two fractions. Table 1 Growth rate constants. Full size table In a second model, we examined the response to treatment, where stationarity/equilibrium is not reached within the observed time period. We used ordinary differential equations (ODEs) to model the joint effect of differential growth and transitions between the two states on the cell population dynamics (Methods): where x L and x H denote the population fraction of efflux Low ( L ) and efflux High ( H ) cells and g i and k i (i=H,L) are the respective rate constants for effective growth and transition, and are separately measured in the absence ( g , k ) and presence ( g′ , k′ ) of the drug ( Table 1 ). As the observed change after 24 h is far from the new equilibrium state and we are only interested in the relative contribution of state transition to the departure from the existing stationary population proportions, we assumed a simple first-order transition, kx . This equation unites the Darwinian and Lamarckian principles, because the effect of selection will come from the difference in g and induction is captured by the difference in k for the two states, in the presence versus absence of the drug ( Table 1 ). Instead of fitting the unknown parameters k H and k L we computed, based on the measured numbers of differential growth rates, how a change of the values for k and g due to the presence of the drug would account for the observed ratio of the two subpopulations, efflux Low and efflux High , at 24 h after administration of VINC, r (24 h)= x H ( t =24 h)/ x L ( t =24 h). The parameter plane ( Fig. 1e ) displays the non-steady state population ratio, r (24 h)=x H / x L after 24 h treatment with VINC, as a function (colour of the map) of the ratios of the growth and state transition rate constants. The almost horizontal course of the colour contour lines, parallel to the x axis that represents variation of the growth parameters g L / g H , indicates that a shift of x H / x L (colour) is minimally affected by the change of the relative growth rate but instead is predominantly defined by a change in the relative state transition rates. Clearly, to achieve the observed appearance of a fraction of 30–40% efflux High cells after 24 h ( Fig. 2a ), corresponding to a ratio x H / x L ≈0.5–0.7 (green zone in parameter space in Fig. 1e ), the measured growth advantage of the efflux High cells in the presence of VINC, at g′ L / g′ H ≈0.25/0.37=0.67, is far from sufficient (dotted vertical line in the parameter space of Fig. 1e ). If there were no cell-individual state transitions, then, with the observed growth differential g′ L / g′ H ( Supplementary Fig. S5 ), selection alone could account for only an increase of MDR High cells to x H / x L =0.04 after 1 day (corresponding to a population fraction of MDR High of ~4%) instead of the observed x H / x L =0.67 (40% MDR High ). The rapid appearance of heterogeneous nuclear RNA (hnRNA) for MDR1 following a 24-h pulse of VINC by targeting the reverse-transcriptase PCR (RT–PCR) to the first intron–exon junction, with a >20-fold induction of MDR1 pre-mRNA at the whole-population level within 30 min of VINC treatment ( Fig. 2b ), followed by detectable expression of mature mRNA followed within 24 h ( Supplementary Fig. S7 ), supports an induction by a molecular change. However, this finding does not prove induction because it could, in principle, reflect an extreme selection of ‘fitter cells’ that display an intrinsic high constitutive synthesis of the MDR1 transcript. Validation of cell-individual induction of resistant state Unequivocal demonstration of cell-individual induction (‘instruction’) of the MDR phenotype requires the direct observation of the actual induction event in the very same cell before and after addition of the drug to the medium by real-time longitudinal monitoring of the cell culture during treatment. The drug-treated cells preloaded with fluorescent dye (efflux Low ) displayed a visible reduction of fluorescence starting 12 h after addition of the drug. In contrast, no change in fluorescence was detectable in the untreated cells. We also observed onset of apoptosis as indicated by DNA condensation in the VINC-treated sample after >24 h ( Fig. 2c and Supplementary Movies 1 and 2 ). Counting after a typical 48-h longitudinal monitoring revealed 63% of the live cells treated with VINC exhibited elimination of the dye, representing the switch to the efflux High phenotype compared with 16% of untreated cells ( n =80 cells; Supplementary Fig. S8 ). To demonstrate that selection per se has no significant role in the emergence of cells with the MDR phenotype, we decoupled MDR1’s functional activity from its expression by blocking MDR1-mediated drug efflux with verapamil [56] , [57] . By separating fitness function of a trait from the expression of that trait, we can expose the role of instructive (non-selective) factors of phenotype change. We first confirmed that baseline or VINC-induced efflux of the fluorescent dye calceinAM (CaAM) was reduced almost completely by saturating doses of verapamil ( Supplementary Fig. S9 ). However, this inhibition of efflux did not measurably suppress the early emergence of the subpopulation of MDR1-expressing cell after VINC treatment ( Fig. 2d ). The observation that cells increased MDR1 expression independently of the increase of the length of pre-incubation with verapamil over the time window in which verapamil gradually unfolds its inhibitory function further suggests that MDR1 induction was independent of the pump function of this protein ( Supplementary Fig. S10 ). This corroborates the role of a selection-independent, instructive mechanism, at least for the rapid appearance of this new phenotype after chemotherapy. This persistent efflux High state induced by a transient drug treatment was also associated with improved survival when the same cells were re-exposed to VINC after washout of the drug ( Fig. 2e ). Thus, drug-induced resistance is non-genetically inherited across cell generations independently of the presence of the drug—at least for a limited period of time ( Supplementary Fig. S11 ). This dynamics represents a Lamarckian scheme for acquisition of a new phenotype. Wnt signalling mediates state transition into a stress state As the presence of discrete efflux High and efflux Low subpopulations may reflect transitions between distinct stable cellular states (attractor states), we next measured their transcriptomes after a 24-h pulse of 10 nM VINC ( Fig. 3a ), when the cell population exhibited a stable bimodal distribution. Even after this short time, globally distinct gene expression pattern were seen when the efflux High and efflux Low subpopulations were compared ( Fig. 3a ). Comparison revealed 974 significantly differentially expressed genes in these two subpopulations, indicating a fractional, globally diverse response within a clonal cell population. Gene Ontology (GO) analysis unveiled the enrichment in this set for genes involved in cell cycle, translation, ribosome and rRNA synthesis, as well as response to DNA damage, metal binding, oxidative phosphorylation and mitochondrial function ( Supplementary Fig. S12 and Supplementary Table S1 ), suggesting that these two transcriptomes represented biologically distinct, high-dimensional attractor states [17] . 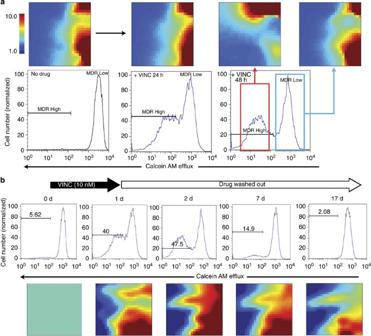Figure 3: EffluxHigh/effluxLowsubpopulations represent distinct functional cell states. (a) Globally distinct transcriptomes of untreated HL60 cells and cells treated with VINC and sorted for effluxHigh/effluxLowdisplayed as self-organized maps with the GEDI programme68. Color bar indicates the log2 of the detection value. Note that effluxLowcells after drug treatment had transcriptomes distinct from that of untreated cells, despite the same MDR status. For full lists of differentially expressed genes, seeSupplementary Data 1. (b) Memory effect of cell state transition after transient drug treatment, indicative of a switch between attractor states. After a transient (24 h) exposure to VINC, the induced MDR phenotype returned to the baseline level after 7–10 days (top), whereas the transcriptome changes persisted until at least day 17 as shown in the GEDI maps (bottom). Here the gene expression was ‘normalized’ to the values at d0, which hence appear in green in the GEDI maps. Figure 3: Efflux High /efflux Low subpopulations represent distinct functional cell states. ( a ) Globally distinct transcriptomes of untreated HL60 cells and cells treated with VINC and sorted for efflux High /efflux Low displayed as self-organized maps with the GEDI programme [68] . Color bar indicates the log2 of the detection value. Note that efflux Low cells after drug treatment had transcriptomes distinct from that of untreated cells, despite the same MDR status. For full lists of differentially expressed genes, see Supplementary Data 1 . ( b ) Memory effect of cell state transition after transient drug treatment, indicative of a switch between attractor states. After a transient (24 h) exposure to VINC, the induced MDR phenotype returned to the baseline level after 7–10 days (top), whereas the transcriptome changes persisted until at least day 17 as shown in the GEDI maps (bottom). Here the gene expression was ‘normalized’ to the values at d0, which hence appear in green in the GEDI maps. Full size image To determine whether a stem-cell-like state has actually been induced by VINC treatment [26] , [40] , [41] , [42] , [43] , [44] , [45] , [46] , [47] , [48] , we next performed pairwise comparisons for all sorted subpopulations, now including untreated cells: cells treated and sorted for efflux High , cells treated and sorted for efflux Low , as well as untreated mock-sorted and treated mock-sorted cells. The set of 2,096 genes that were significantly expressed above background (BeadChip detection p-value<0.05, Methods), and whose expression level differed for each comparison pair by more than fourfold, were first manually examined for the relevant functional annotations using the NCBI Gene database and the stem-cell signatures reported in Brandenberger et al . [58] Of note are the alterations in the expression of genes that belong to the Wnt and Polycomb pathways, consistent with the role of a stemness signature in drug-resistant tumour cells. These differentially expressed genes were also subjected to unbiased gene set enrichment analysis (GSEA; Supplementary Fig. S13 ), which also extracted the Wnt signalling [59] gene set ( Supplementary Figs S14 and S16 ) in line with previous studies [60] , [61] , showing an apparent ‘induction’ of Wnt during therapy. Many of the gene expression changes induced by VINC treatment were not detected when we simply compared treated and untreated whole (not sorted) cell cultures, highlighting the cell population heterogeneity and the importance of cell sorting to isolate relevant cell subpopulations for biochemical cell analysis. A feature of a high-dimensional attractor state is the memory of the perturbation, that is, a lasting change of a large set of responding genes that persists after removal of the perturbation. To determine whether the transcriptome-wide adaptive response exhibited such memory, VINC was washed out after the 24 h treatment. Whereas the efflux High phenotype persisted for a week after transient exposure to VINC ( Fig. 3b ), the VINC-treated cells remained globally altered beyond 17 days, long after the population had relaxed to the native distribution with baseline efflux ( Fig. 3b and Supplementary Fig. S15 ). Crucially, if the reappearance of the efflux Low state, which has a growth advantage in the absence of drug ( Supplementary Fig. S5 ), is the result of selection of naive efflux Low cells (which either have never responded or fully reverted back), one would expect to see the reappearance of the transcriptome of untreated cells. However, in these post-treatment cells, the global changes in gene expression triggered by VINC persisted for >17 days, suggesting that VINC induced an adaptive, slowly reversible response with respect to the efflux phenotype as a non-specific stress response, but a stable (apparently irreversible) attractor transition with respect to other state space dimensions, which are orthogonal to those conferring the efflux phenotype. As many Wnt pathway components ( Supplementary Fig. S16 ) were highly induced in the efflux High cells, we next knocked down β-catenin in HL60 cells to determine whether it has an active role in the induction of the MDR phenotype ( Supplementary Fig. S17 ). When β-catenin was suppressed, after 60h of VINC treatment both efflux capacity ( Fig. 4a ) and MDR1 expression ( Fig. 4b ) were reduced by half relative to the control. This inhibition had functional consequences, because the viability of β-catenin knockdown cells in just 1 nM VINC was reduced to half compared with the control ( Fig. 4c ). Rescue by ectopic overexpression of an RNA interference-resistant β-catenin construct completely restored VINC-induced efflux and expression of MDR1 in the knockdown cells, confirming specificity of the knockdown ( Supplementary Fig. S18 ). 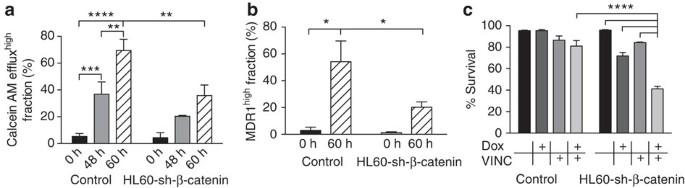Figure 4: Inhibition of β-catenin suppresses drug-induced resistance and MDR1 expression. CalceinAM efflux (a) and MDR1 expression (b) induction in HL60 cells by VINC (1 nM VINC) at indicated times are suppressed when β-catenin is knocked down using a lentiviral doxycycline (dox) -inducible small hairpin RNA construct (sh-β-catenin). This suppression of the Wnt pathway also compromised viability of the cells in the presence of low VINC concentrations (*, **, *** and **** denote comparisons withP-value <0.05, 0.01, 0.001 and 0.0001, respectively (two-way analysis of variance); error bars, s.d.,n=three biological replicates from one representative of three independent experiments performed in two different laboratories). Figure 4: Inhibition of β-catenin suppresses drug-induced resistance and MDR1 expression. CalceinAM efflux ( a ) and MDR1 expression ( b ) induction in HL60 cells by VINC (1 nM VINC) at indicated times are suppressed when β-catenin is knocked down using a lentiviral doxycycline (dox) -inducible small hairpin RNA construct (sh-β-catenin). This suppression of the Wnt pathway also compromised viability of the cells in the presence of low VINC concentrations (*, **, *** and **** denote comparisons with P -value <0.05, 0.01, 0.001 and 0.0001, respectively (two-way analysis of variance); error bars, s.d., n =three biological replicates from one representative of three independent experiments performed in two different laboratories). Full size image Our analysis of the rapid ‘appearance’ of the MDR phenotype and of MDR1 expression following chemotherapy provides evidence that this early drug resistance phenotype can be induced by a Lamarckian instruction, independent of selection. Our conclusion is supported by a series of findings: first, the experimental measurement of a rapid drug-triggered induction of a MDR1 High (efflux High ) subpopulation comprising 40% of the cells within 1 day and associated mathematical cell population dynamics modelling show that the observed moderate fitness advantage of the efflux High cells cannot account for this response kinetics. Second, single-cell longitudinal monitoring directly demonstrates ‘true’, cell-individual adaptation. Third, the decoupling of the expression of a trait from its function (which conveys selective advantage) excludes a role for Darwinian selection. Finally, transcriptome analysis reveals a genome-wide, distinct and enduring stress-induced state that is unlikely orchestrated by random mutations. The results of course do not preclude a role of canonical Darwinian somatic evolution driven by the selection of random genetic mutants at later stages, as amply supported by the observed genomic alterations whose nature readily offer a mechanistic rationale for selective advantage. However, the argumentation for this evolutionary scheme as the sole mechanism requires the assumption of a substantial amount of pre-existing mutations [11] . This requirement is alleviated by admitting non-genetic processes as a catalyser [31] , [32] , which is mediated by cells that either transiently, and by chance, occupy a stem-like attractor state and hence survive the treatment, or are induced by the cytotoxic stress to enter such a protective state. Here we show that the latter dominates. Although the apparent ‘activation’ of resistance mechanisms and alternative survival pathways or of stem-like states after drug or radiation therapy is frequently observed [26] , [40] , [41] , [42] , [43] , [44] , [45] , [46] , [47] , [48] , the distinction between Lamarckian induction and Darwinian selection is rarely explicitly articulated. Existing thinking in cancer biology tacitly implies the latter but often communication is blurred by the use of metaphoric shorthand expressions that are common in evolution biology, such as the ‘the tumour adapts to the therapy’, which suggests the former. Awareness of this dualism and specifically, of non-genetic dynamics may help to explain several non-intuitive tumour behaviours, such as follows: why does treatment not only cause drug resistance but inseparably also increases malignancy in recurrent tumours; why can drug resistance not be suppressed by just blocking MDR1 (ref. 57 ); why do early tumour cell clones disappear and reappear [62] or why do recurrent tumours, after developing resistance to target-selective drugs, become sensitive to the same therapy again [63] , [64] . Considering non-genetic and drug-triggered cell-state dynamics may open new opportunities for the management of resistant tumours, such as targeting molecular pathways before conventional treatment to prevent therapy-induced tumour progression. Cell culture Acute leukemic cell line HL60 was obtained from ATCC, and independently re-cloned twice from individual cells and cultured in three independent laboratories (see author affiliations). HL60 cells were cultured in Iscove’s modified Dulbecco’s medium (Invitrogen) supplemented with 20% fetal bovine serum (Sigma), 1% L -glutamine, penicillin (100 U ml −1 , Invitrogen) and streptomycin (100 mg ml −1 , Invitrogen). Cell number was monitored daily and culture was maintained at a density of 2 × 10 5 to 2 × 10 6 cells per ml. Viable cell count To determine the viability and number of cells, 0.4% trypan blue solution was used. Cell suspensions were diluted 1:5 with trypan blue and viable cells, which exclude the dye, were scored on a haemocytometer under a light microscope. Flow cytometry HL60 cells were labelled with MDR1/P-glycoprotein APC-conjugated mouse anti-human monoclonal antibody (e-Biosciences, 2.5 ng μl −1 ). Flow cytometry analysis was performed on a BD FACSCalibur cell cytometer or a Guava cell cytometer. To determine the percentage of labelled cells, a quadrant gate using an equal concentration of a relevant mouse isotype control was placed. For each analysis, 10,000 of viable events that exclude Propidium Iodide (PI, Sigma) were saved. For cell cycle studies, cells were labelled with 1 mM DRAQ5 (Axxora, San Diego, CA) according to manufacturer’s instructions. MDR functional assay HL60 cells (2 × 10 5 ) were washed in Hank’s balanced salt solution/5% fetal bovine serum (washing buffer) and then incubated with 1 nM of CaAM (Invitrogen) for 15 min at 37 °C. Cells were then washed in cold buffer and resuspended in PI staining buffer (PI in washing buffer, 1:200 dilution), and samples were kept on ice until analysis. For each analysis in the cytometer, 10,000 of viable events that exclude PI were saved. As controls, cells that had not been loaded with CaAM were used. In addition, dead cells were also gated out using scatter characteristics. Fluorescence-activated cell sorting FACS analysis was conducted on a BD Biosciences Aria II at the Hematologic Neoplasia Flow Cytometry Facility of the Dana Farber Cancer Institute. For studies of the dynamics of sorted subpopulations, antibodies (2.5 ng μl −1 ) were removed following cell sorting using brief incubation in low-pH buffer [29] . RNA isolation Approximately 7–10 × 10 6 cells were collected for RNA isolation from each condition or subpopulation. RNA was extracted following standard protocol from RNeasy Mini Kit (Qiagen). Quantitative RT–PCR Two hundred nanograms of total cellular RNA was used to prepare complementary DNA following the standard protocol from iScript cDNA synthesis kit (BioRad). QuantitativePCR analysis was performed according to the manufacturer’s protocol using iTaq SYBR Green Supermix with Rox (BioRad). Three hundred nanomolars each of forward and reverse MDR1 primers were used. MDR1 primer sequences were as follows: for the hnRNA(Ex1–Intr1): 5′-CTCACTTCAGGAAGCAACCA-3′ (forward) and 5′-TGATTGCAAACTTCTAGTCAAGACA-3′ (reverse); for the hnRNA(Intr1–Ex2): 5′-TGGAGAGGTCGGAGTTTTTG-3′ (forward) and 5′-GGTTGAATTTCCAGGAGGAATG-3′ (reverse); for the coding region: 5′-TACAGTGGAATTGGTGCTGGG-3′ (forward) and 5′CCCAGTGAAAAAATGTTGCCA-3′ (reverse). Quantitative RT–PCR was carried out with a BioRad CFX96 real-time system C1000 and the iQ5 thermal cycler. Single-cell imaging HL60 cells were labelled with CaAM using the Vybrant Multidrug Resistance Assay or 10 μg ml −1 of Rhodamine123 (Rh123, Invitrogen). Single cells were seeded into 96-well optical plates with a BD FACS Aria (Dana Farber Hematologic Neoplasia Core Facility) based on size/forward scatter, regardless of CaAM fluorescence. Following plating, a baseline fluorescence image was obtained for each individual cell. Ten nanomolars VINC or an equivalent volume of drug-free control media was added to each well and the dye pumping function of individual cells was measured by imaging CaAM fluorescence 24 and 48 h after drug administration. Phase-contrast imaging was conducted in parallel to assist in locating the cell within the well. Live-cell microscopy HL60 cells at a density of 1 × 10 6 cells ml −1 were seeded for 30 min in a glass-bottom dish (Iwaki) and imaged with a Zeiss Exciter (Plan-Neofluar × 40 NA 1.3 Oil DIC). Cells were stained with Rh123 (Invitrogen; 1:20,000) or Hoechst 33342 (Invitrogen; 1:200,000). For both dyes, the expression level was monitored until it reached a plateau (uptake) before initiation of experiment. Image analysis was conducted with LSM Aim Software. β-catenin constructs β-catenin small hairpin construct: β-catenin targeting small hairpin (shRNA) was kindly provided by Jürgen Deka. It was cloned using a published β-catenin target sequence [65] . The oligonucleotide was subcloned ( Xho 1 and Eco R1) into the pInducer11 backbone (kindly provided by Stephen Elledge [66] ) to result in pInd-β-catenin. shRNA-resistant β-catenin. An shRNA-resistant β-catenin cDNA was kindly provided by Jürgen Deka and Frédérique Baruthio. It is based on a β-catenin D164A plasmid [67] , which was kindly provided by Konrad Basler. The D164A mutation was reversed by PCR. The pInd-β-catenin construct targets the following sequence (underlined) in β-catenin: (1,580 bp) 5′-GTCTGCCAA GTGGGTGGTATAGAGGCTC TTGTGCGTACTGTCCTTCGGGCT-3′ (1,630 bp). Wobble base mutations were introduced under consideration of highest human codon usage into the target sequence (underlined), resulting in a rescue cDNA fragment: 5′-GT C GG A GGCAT T GA A GC C C-3′. The β-catenin rescue fragment was amplified by PCR using AttB-containing primers and subsequently subcloned into pInducer20 (kindly provided by Stephen Elledge [66] ) resulting in pInd-β-cat-rescue. Western blot analysis HL60 parental cells, sh-β-catenin knockdown cells and rescued (sh-resistant cDNA) knockdown cells were cultured in regular growing medium supplemented with 2 μg ml −1 doxycycline for 96 h. Cells (10 7 ) were suspended in CelLytic MT cell lysis reagent (Sigma-Aldrich) containing protease inhibitors (Complete mini cocktail, Roche). The lysis solution was sonicated and centrifuged, and the total protein extraction contained in the supernatant was quantified based on the Bradford colorimetric assay (BioRad). Samples were resolved by electrophoresis on a 8% SDS–PAGE gel, transferred to a polyvinylidene difluoride membrane and probed with primary antibodies against β-catenin (1:2,000 in TBST +5% BSA; BD Biosciences) and α-Tubulin (loading control, 1:3,000 in TBST; Calbiochem). A horseradish peroxidase-conjugated goat anti-mouse antibody was added, and secondary antibodies were detected through chemiluminescence (ECL, Amersham) on a Fusion FX7 charge-coupled device image acquisition system. Statistical analysis Two-way analysis of variance followed by Dunnett’s multiple comparisons test was performed using GraphPad Prism version 6.00 for MacOS, GraphPad Software, La Jolla, CA USA, www.graphpad.com . Mathematical modelling For the Markov state transition model, we make two assumptions. First, we discretize the continuous distribution of cell population as two discrete states, MDR Low and MDR High . This is warranted given the bimodal distribution (that is better visible in the drug-induced conditions). Second, we assume that the probabilities at each time step for staying in the same state (‘self-renewal’) and for transition are linear (first-order kinetics). The governing equations of the Markov model of the state transition model are (equation 2): where denote the initial relative proportions of cells in the two respective states MDR Low ( L ) and MDR High ( H ) and represent the relative proportions of cells in the MDR Low and MDR High states in the n −the time step ( x L + x H =1). P ij represents the probabilities of transitioning from state i to j (the basis of instruction by the drug) and P ii represents the ‘self-renewal’ (probability of staying in the same state), as previously employed [21] , although the Markov mode is not a growth model. Because of its Markov property, the transition matrix P satisfies: It also has a maximum eigenvalue and a corresponding eigenvector, which determines the final steady state of cell population. With this equation, we can study the influence of the transition rates and the self-renewal rates on the steady state. From equation(4), we obtain for the steady-state ratio r* = x* L /x* H of the two populations, efflux Low and efflux High : With this model, we determine the parameter space, which maps the relative values of growth and transition rates to a given steady-state composition, r* . Using the numbers for the observed effective growth rate constants ( g L , g H ; Table 1 ) in equation(5) for the relative magnitudes of P LL and P HH , we display r* as a function of the ratios of the transition rates P LH and P HL , and of the self-renewal rates P LL and P HH on the steady-state ratio r* ( Fig. 1d ). One cannot measure the effective transition rates accurately, because the observed apparent reconstitution of the efflux High population from the sorted efflux Low cells is a composite result of effective transition and effective growth, and the observed state transition is slower than cell proliferation. By contrast, the initial effective growth rates of the sorted subpopulations can be reliably estimated, because in this initial period the transition to and from the other state is negligible for both subpopulations due to the small probabilities P or the small population size n . For the Linear ordinary differential equation model a s with the Markov model, we discretize the continuous distribution of cell population as two distinct states, MDR Low and MDR High , and assume again that the rate of both cell effective growth (death and birth combined) and transitions follow first-order kinetics. The governing equations of the linear ODE model can be written as follows (equation 6): where x L and x H denote the population fraction of efflux Low ( L ) and efflux High ( H ) cells as in the last Markov model. g i and k i (i=H,L) are the respective rate constants for effective growth and transition, and are separately measured for absence ( g , k ) and presence ( g′ , k′ ) of the drug. The mathematical solutions of equation (6) depend on the eigenvalue of following matrix: With the quadratic equation for the eigenvalue λ and the solutions λ 1 and λ 2 , the solution of the ODEs is: We numerically estimated the ratios of growth rate constants and the transition rate constants , which produce a given ratio of the subpopulations r (24 h)= x H (24 h)/ x L (24 h) after 24 h of drug treatment as displayed in Fig. 1e using the values shown in the Table 1 . Microarray analysis Microarray studies were performed by the Molecular Genetics Core Facility at Children’s Hospital Boston supported by NIH-P50-NS40828 and NIH-P30-HD18655. RNA samples were hybridized to Illumina Human Ref-3 expression BeadChips, and initial processing and normalization was performed with BeadStudio software. BeadChip internal P -values (technical bead replicates) were used for filtering out genes significantly expressed above the background noise. To filter out genes with signals not significant above the background noise, P -value from Illumina BeadStudio (see above) of 0.05 was used as the cutoff value and only genes with a P -value <0.05 in all four samples passed the filter. From the original set of 18,401 probes, 2,096 genes met this criterion. Significant genes were identified with Significance Analysis of Microarrays using a false-discovery rate of <1% on all genes, resulting in 974 genes. Self-organized maps of significant gene lists were prepared using the Gene Expression Dynamics Inspector software ( http://www.childrenshospital.org/research/ingber/GEDI/gedihome.htm ) [68] . Hierarchical clustering based on Euclidean distance was performed on time course gene expression data normalized by z- score. Gene expression data have been deposited in the GEO databank under this publication ID. For GSEA, the data set analysed corresponds to the four samples shown in Fig. 3 (MDR-High subpopulation after VINC (sample 1); MDR-Low subpopulation after VINC (sample 2); no treatment/mock sort, (sample 3); and VINC treatment/mock sort (sample 4). The gene set with 2,096 genes (see above) was normalized using the quantilenorm function in MatLab. The aim was to identify genes differentially expressed between the untreated population (sample 3) and the other three samples. To do that, we calculated the pairwise ratios between sample 3 and samples 1, 2 and 4, respectively. Genes with a log fold change (log2(ratio)) ≥2 or ≤−2 are listed in Supplementary Data 1 . The genes in Supplementary Data 1 , columns 2 (sample 3 versus sample 2) and column 3 (sample 3 versus sample 4), were manually checked for their biological function using NCBI–Gene database. For the genes listed in Table 1 column 1 (sample 3 versus sample 1), we manually mapped it to the stemness pathways identified by Branderberg et al . [58] The set of 2,096 genes was subjected to GSEA [69] to identify gene sets in MSigDB enriched for genes of KEGG (Kyoto Encyclopedia of Genes and Genomes) pathways in all the samples when using untreated mock-sorted samples as reference ( Supplementary Fig. S14 ). A ranked list is presented as a heat map plot in Supplementary Fig. S13 , showing the most significantly differentially expressed genes between mock-sorted and the other three samples (treated/mock-sorted, treated/sorted low efflux, treated/sorted high efflux). The GSEA analysis expands the manual approach and confirms the stem-cell signature of the Wnt pathway, whose genes are differentially expressed after treatment. For GO analysis, the same gene set used for GSEA was tested in DAVID (Database for Annotation, Visualization and Integrated Discovery) against the Homo sapiens gene reference set [70] . Sixteen functional categories were found to be significantly enriched in the data set with a P -value<0.001. These GO terms, their significance and the number of associated genes in the data set are summarized in Supplementary Table S1 . Accession codes : Sequence data have been deposited in GEO under accession number GSE49869 . How to cite this article: Pisco, A.O. et al . Non-Darwinian dynamics in therapy-induced cancer drug resistance. Nat. Commun. 4:2467 doi: 10.1038/ncomms3467 (2013).